Selective conversion of CO2and H2into aromatics Transformation of greenhouse gas CO 2 and renewable H 2 into fuels and commodity chemicals is recognized as a promising route to store fluctuating renewable energy. Although several C 1 chemicals, olefins, and gasoline have been successfully synthesized by CO 2 hydrogenation, selective conversion of CO 2 and H 2 into aromatics is still challenging due to the high unsaturation degree and complex structures of aromatics. Here we report a composite catalyst of ZnAlO x and H-ZSM-5 which yields high aromatics selectivity (73.9%) with extremely low CH 4 selectivity (0.4%) among the carbon products without CO. Methanol and dimethyl ether, which are synthesized by hydrogenation of formate species formed on ZnAlO x surface, are transmitted to H-ZSM-5 and subsequently converted into olefins and finally aromatics. Furthermore, 58.1% p -xylene in xylenes is achieved over the composite catalyst containing Si-H-ZSM-5. ZnAlO x &H-ZSM-5 suggests a promising application in manufacturing aromatics from CO 2 and H 2 . The utilization of fossil resources such as coal, oil, and natural gas has brought us unprecedented economy and social development in the past two centuries [1] , however, continuously increasing the emissions of greenhouse gas CO 2 is threatening our living environment. The renewable energy resources (for example, solar, tidal, wind and biomass) can generate abundant power, but low-efficiency and fluctuating nature limits their widespread applications [2] . These problems above could be effectively overcome via CO 2 hydrogenation to fuels (e.g., gasoline) and commodity chemicals (e.g., methanol, olefins and aromatics) because hydrogen can be acquired from the clean electricity [3] , [4] , [5] , [6] . Considering that CO 2 (Δ f G o = −396 kJ mol −1 ) is a chemical inert molecular [3] , CO 2 hydrogenation reactions are generally operated under high pressure and hydrogen content over reductive metal catalysts so as to improve the conversion efficiency. Nowadays, C 1 chemicals such as methanol (MeOH), dimethyl ether (DME), formic acid (HCOOH), methane (CH 4 ), and carbon monoxide (CO) have been selectively synthesized under above conditions [3] , [4] , [6] , [7] . However, production of C 2+ hydrocarbons such as olefins and liquid fuels from CO 2 are not easy because of high kinetic barriers for C–C coupling [6] , [8] . In the earlier studies, combination of reverse-water-gas-shift (RWGS, CO 2 + H 2 → CO + H 2 O) and Fischer–Tropsch (FT, CO + H 2 → C n H m ) synthesis reactions was considered as a promising method to generate long-chain hydrocarbons from CO 2 [2] , [9] . Nevertheless, due to the restriction of Anderson–Schulz–Flory (ASF) distribution [10] , [11] , the selectivity of C 2 –C 4 and gasoline fraction hydrocarbons does not exceed 58% and 48% [12] , [13] , respectively. More recently, high selective olefins or gasoline has been achieved from CO 2 hydrogenation via utilization of oxide/zeolite bifunctional catalysts which have been successfully applied in syngas-to-olefins (STO) or aromatics (STA) reactions [14] , [15] , [16] , [17] , [18] , [19] , [20] . Some typical results are as follows: In−Zr oxide, ZnGa 2 O 4 or ZnO-ZrO 2 combined with SAPO-34 zeolites achieved more than 80% C 2 –C 4 olefins [21] , [22] , [23] , meanwhile, In 2 O 3 or Na-Fe 3 O 4 coupled with H-ZSM-5 zeolites reached to approximately 80% gasoline-range hydrocarbons [24] , [25] . Because metal catalysts or the Brønsted acid sites of the zeolites can catalyze hydrogenation reactions [26] , [27] , it is challenging to synthesize aromatics with high unsaturation degree and complex structures under conditions of high H 2 content. Up to now, there are no reports on the highly selective conversion of CO 2 and H 2 into aromatics. Here, we report a composite catalyst made by nano-scaled spinel structural ZnAlO x oxide and H-ZSM-5 zeolite (ZnAlO x &H-ZSM-5), which exhibits 73.9% aromatics selectivity with only 0.4% CH 4 selectivity among the carbon products without CO in CO 2 hydrogenation reaction. RWGS reaction is largely suppressed by increasing H 2 /CO 2 ratio or introducing CO. 58.1% p -xylene in xylenes is achieved over the composite catalyst containing Si-H-ZSM-5. Reaction mechanism and the causes of excellent aromatization performance are also explored. Catalytic results CO 2 hydrogenation reactions were conducted over ZnAlO x &H-ZSM-5 under reaction conditions of H 2 /CO 2 /Ar = 3/1/0.2, pressure 3.0 MPa, and 593 K. The effects of space velocity on CO 2 conversion and product selectivity are shown in Fig. 1a . It is surprising to find that the selectivity of aromatics among the carbon products without CO reaches as high as 73.9% with 9.1% CO 2 conversion and 57.4% CO selectivity at space velocity = 2000 ml g −1 h −1 . This aromatics selectivity is much higher than the about 40% obtained over Na-Fe 3 O 4 /H-ZSM-5 [25] or 14.6% acquired over In 2 O 3 /H-ZSM-5 [24] , respectively. Besides that, the liquid (or gasoline-range) hydrocarbons including C 5+ and aromatics (excluding CO) run up to 80.3% along with merely 0.4% CH 4 . As the space velocity substantially rises to 10,000 ml g −1 h −1 , the aromatics selectivity only slightly decreases to 56.9%. This result is quite different from STA reactions, which were often operated at the GHSV <1500 ml g −1 h −1 so as to peruse high aromatics selectivity [19] , [20] . It also can be seen from Fig. 1a that MeOH, DME and C 2-4 olefins are progressively climbing with the space velocity growing, which suggests that these byproducts might be acted as the intermediates for aromatization. The CO 2 hydrogenation behaviors of various catalysts are compared in Fig. 1b . ZnO exhibits 98.2% MeOH selectivity (excluding CO) with 2.6% CO 2 conversion and 63.5% CO selectivity. After mixed with H-ZSM-5, only 29.7% aromatics selectivity was achieved. Compared to ZnO, ZnAlO x shows a higher CO 2 conversion (5.1%) but lower CO selectivity (54.9%). The DME and MeOH selectivity is up to 42.8% and 56.2% over ZnAlO x , respectively. It implies that AlO x component is acted as the active site for MeOH dehydration. In contrast with the composite catalyst ZnO&H-ZSM-5, the composite catalyst ZnAlO x &H-ZSM-5 shows a much better aromatization performance, over which 66.2% aromatic selectivity is obtained under the same reaction conditions. As shown in Fig. 1b , although the CO 2 conversion and liquid hydrocarbons selectivity are approximate, the aromatics selectivity for ZnAlO x &H-ZSM-5 prepared by two components grinding in an agate mortar is 12.4% higher than ZnAlO x + H-ZSM-5 prepared by the granules of two components mixing. It is apparent that the proximity of oxides and zeolites for the former catalyst is better than the latter one. It means that the closer proximity favors the selective generation of aromatics. As a comparison, the dual-bed configuration catalyst ZnAlO x /H-ZSM-5 with H-ZSM-5 downstream from the ZnAlO x provided the poorest behavior with 17.9% aromatics selectivity. The effect of reaction temperature on the CO 2 hydrogenation over ZnAlO x &H-ZSM-5 is investigated. Although raising temperature can increase the CO 2 conversion, the ability of aromatization is considerably weakened (Supplementary Fig. 1 ). The optimized weight ratio of oxide/zeolite is 1:1 (Supplementary Fig. 2 ). We also studied the CO 2 hydrogenation over the mixture of conventional methanol synthesis catalyst CuZnAlO x and H-ZSM-5. As shown in Supplementary Fig. 3 , the RWGS reaction is predominant, which leads to more than 95% CO selectivity. According to the conditions for CO 2 hydrogenation, CO hydrogenation over ZnAlO x &H-ZSM-5 was investigated at H 2 /CO/Ar = 3/1/0.2, space velocity = 6000 ml g −1 h −1 , pressure 3.0 MPa, and 593 K. As depicted in Supplementary Fig. 4 , the aromatics selectivity (excluding CO 2 ) is only 12.8% with 4.7% CO conversion. It implies that the excellent aromatization behavior of ZnAlO x &H-ZSM-5 in CO 2 hydrogenation is not related to self-promotion mechanism of CO reported by Cheng et al. [19] . Fig. 1 Catalytic performance for CO 2 hydrogenation. a The effect of space velocity over ZnAlO x &H-ZSM-5. Reaction conditions: 593 K, 3.0 MPa, H 2 /CO 2 /Ar = 3/1/0.2. b Comparisons of the CO 2 conversion and product selectivity over various catalysts. Reaction conditions: Space velocity = 12,000 (for ZnO and ZnAlO x ) or 6000 (for composite catalysts) ml g −1 h −1 , 3.0 MPa, 593 K, H 2 /CO 2 /Ar = 3/1/0.2. Note that the C 5+ excludes aromatics. C 2-4 = and C 2-4 o refer to C 2 –C 4 olefins and paraffins, respectively; ZnAlO x &H-ZSM-5 prepared by grinding; ZnAlO x + H-ZSM-5 prepared by granules mixing; ZnAlO x /H-ZSM-5 denoted as dual-bed catalysts Full size image Catalytic stability The catalytic stability of ZnAlO x &H-ZSM-5 in CO 2 hydrogenation reaction was studied. It is apparent from Fig. 2 that the composite catalyst delivers a good stability in a 100 h test. The CO 2 conversion, liquid hydrocarbons, and CH 4 selectivity among the carbon products without CO levels off at around 5.4, 74.0, and 0.5% after 50 h on stream. Although the aromatics selectivity is slightly decreased from 72.0% in the initial state to 66.0% after 100 h on stream, the formation rate of aromatics can keep about 15 mg g −1 h −1 because the CO selectivity progressively declines. Fig. 2 The stability test for CO 2 hydrogenation over ZnAlO x &H-ZSM-5. Reaction conditions: Space velocity = 6000 ml g −1 h −1 , 3.0 MPa, 593 K, H 2 /CO 2 /Ar = 3/1/0.2. Note that the liquid hydrocarbons include aromatics Full size image Selectivity optimization In order to improve the efficiency for CO 2 hydrogenation to valuable hydrocarbons such as aromatics, light olefins and gasoline, the RWGS reaction should be suppressed as much as possible. It is very interesting to find from Fig. 3a that as the H 2 /CO 2 ratio rises from 3/1 to 9/1, the CO 2 conversion is dramatically increased from 5.8 to 15.7% with the CO selectivity sharply decreasing from 56.9 to 28.7%. It means that the generated CO can be further converted by hydrogenation in the high H 2 /CO 2 ratio. Although raising H 2 /CO 2 ratio can slightly decrease aromatics selectivity, their formation rate keeps growing. Further increasing H 2 /CO 2 ratio to 15/1 leads to a decline in aromatization rate. Moreover, the liquid hydrocarbons are not sensitive to H 2 /CO 2 ratio. As shown in Fig. 3b , another effective method to weaken RWGS reaction is adding CO into the mixture gas of CO 2 and H 2 . The CO selectivity is nearly monotonically decreasing with CO/CO 2 ratio increasing and as low as 12.6% at CO/CO 2 ratio = 1.8/1, nevertheless, the aromatics or liquid hydrocarbons selectivity is slightly influenced after CO introduction. As known, RWGS is a typical equilibrium reaction [4] . Therefore, introduction product CO does not benefit the formation of itself. These results above are vital to applications. On the one hand, the source of feed gas is more extensive because its composition can be adjusted in a wide range; on the other hand, the product CO can be recycled and accumulated so as to practically depress the RWGS reaction. As presented in Fig. 3c , aromatics with 9 to 10 carbons are predominant over ZnAlO x &H-ZSM-5. We tried to optimize the distributions of aromatics by using Si-H-ZSM-5 made by tetraethoxysilane (TEOS) modification. Compared to ZnAlO x &H-ZSM-5, ZnAlO x &Si-H-ZSM-5 obviously produces more toluene (2.7%) and xylenes (16.8%) (Fig. 3c ). Moreover, 58.1% p -xylene in xylenes, 25.3% ethylene and 11.9% propylene (excluding CO) along with little C 1-3 alkanes are obtained over ZnAlO x &Si-H-ZSM-5 (Fig. 3c and Supplementary Fig. 5 ). The catalytic behavior for ZnAlO x &Si-H-ZSM-5 would be interesting to industry, because ethylene, propylene and p -xylene are the most important commodity hydrocarbon chemicals. Fig. 3 The results of selectivity optimization for CO 2 hydrogenation. a The effect of H 2 /CO 2 ratio over ZnAlO x &H-ZSM-5. Reaction conditions: Space velocity = 6000 ml g −1 h −1 , 3.0 MPa, 593 K. b The effect of CO introduction over ZnAlO x &H-ZSM-5. Reaction conditions: catalyst weight = 667 mg, 3.0 MPa, 593 K, inlet gas containing 66.7 ml min −1 mixed gas (H 2 /CO 2 /Ar = 3/1/0.2) and 0–26.6 ml min −1 CO. c Comparisons of catalytic behaviors over ZnAlO x &H-ZSM-5 and ZnAlO x &Si-H-ZSM-5. Reaction conditions: Space velocity = 6000 ml g −1 h −1 , 3.0 MPa, 593 K, H 2 /CO 2 /Ar = 3/1/0.2. A9 and A10 are representative of aromatics containing 9 and 10 carbon atoms, respectively Full size image Structural characterization Figure 4a shows the X-ray diffraction (XRD) patterns of ZnAlO x oxide. The reflection peaks of ZnAlO x can be approximately assigned to cubic ZnAl 2 O 4 gahnite [28] (JCPDS 05-0669, Supplementary Fig. 6 ). 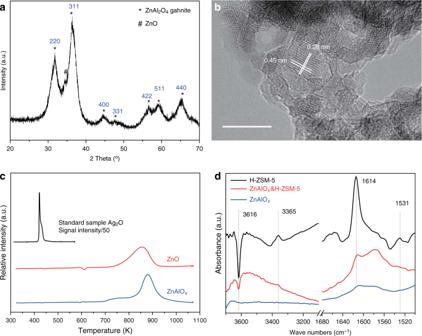Fig. 4 Structural characterization of various catalysts.aX-ray diffraction patterns (XRD) of ZnAlOx.bHigh-resolution transmission electron microscopy (TEM) image of ZnAlOx. Scale bar: 10 nm.cH2-TPR profiles. The relative intensity was normalized by weight. The relative intensity of the standard sample Ag2O was divided by 50.dFTIR subtraction spectra relative to adsorption of DTBPy The reflection peaks of ZnO (Supplementary Fig. 7 ) are hardly detectable for ZnAlO x . The Field-emission scanning electron microscopy (SEM) image (Supplementary Fig. 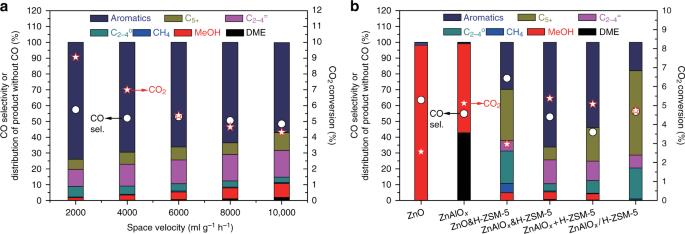8 ) shows that the morphology of ZnAlO x is porous and made by small particles. Fig. 1 Catalytic performance for CO2hydrogenation.aThe effect of space velocity over ZnAlOx&H-ZSM-5. Reaction conditions: 593 K, 3.0 MPa, H2/CO2/Ar = 3/1/0.2.bComparisons of the CO2conversion and product selectivity over various catalysts. Reaction conditions: Space velocity = 12,000 (for ZnO and ZnAlOx) or 6000 (for composite catalysts) ml g−1h−1, 3.0 MPa, 593 K, H2/CO2/Ar = 3/1/0.2. Note that the C5+excludes aromatics. C2-4=and C2-4orefer to C2–C4olefins and paraffins, respectively; ZnAlOx&H-ZSM-5 prepared by grinding; ZnAlOx+ H-ZSM-5 prepared by granules mixing; ZnAlOx/H-ZSM-5 denoted as dual-bed catalysts The BET surface area of ZnAlO x (Supplementary Table 1 ) is up to 151.0 m 2 g −1 , which is much higher than ZnO (11.9 m 2 g −1 ). High-resolution transmission electron microscopy (TEM) image in Fig. 4b gives us the fact that the ZnAlO x sample consists of a lot of tiny nanoparticles with the sizes of <10 nm. Moreover, the lattice spaces of 0.28 and 0.45 nm which respectively correspond to the (220) and (111) planes of cubic ZnAl 2 O 4 further confirm the spinel structure of ZnAlO x [28] . The element distribution analysis (Supplementary Fig. 9 ) shows that the Zn, Al, and O are uniformly dispersed. As presented in Supplementary Fig. 10 , the ZnO sample in this study is consisted of about 100 nm nanoparticles with a clear lattice space. The H-ZSM-5 zeolite embraces a typical nano-sized MFI structure (Supplementary Fig. 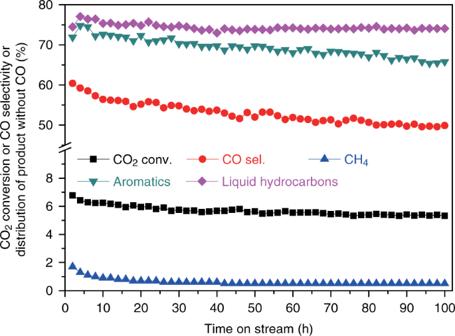11 ). Fig. 2 The stability test for CO2hydrogenation over ZnAlOx&H-ZSM-5. Reaction conditions: Space velocity = 6000 ml g−1h−1, 3.0 MPa, 593 K, H2/CO2/Ar = 3/1/0.2. Note that the liquid hydrocarbons include aromatics The acidcontent of H-ZSM-5 is 1.3 times as high as Si-H-ZSM-5 (Supplementary Table 2 ). 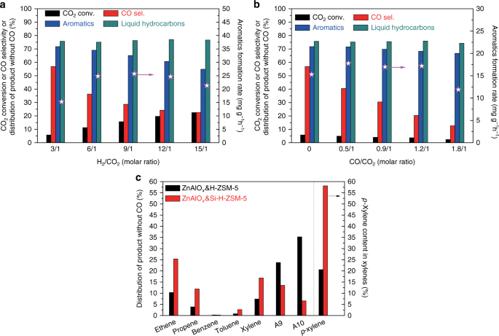The temperature-programmed reduction (TPR) results in Fig. Fig. 3 The results of selectivity optimization for CO2hydrogenation.aThe effect of H2/CO2ratio over ZnAlOx&H-ZSM-5. Reaction conditions: Space velocity = 6000 ml g−1h−1, 3.0 MPa, 593 K.bThe effect of CO introduction over ZnAlOx&H-ZSM-5. Reaction conditions: catalyst weight = 667 mg, 3.0 MPa, 593 K, inlet gas containing 66.7 ml min−1mixed gas (H2/CO2/Ar = 3/1/0.2) and 0–26.6 ml min−1CO.cComparisons of catalytic behaviors over ZnAlOx&H-ZSM-5 and ZnAlOx&Si-H-ZSM-5. Reaction conditions: Space velocity = 6000 ml g−1h−1, 3.0 MPa, 593 K, H2/CO2/Ar = 3/1/0.2. A9 and A10 are representative of aromatics containing 9 and 10 carbon atoms, respectively 4c and Supplementary Table 3 show that both of ZnAlO x and ZnO can be hardly reduced by H 2 below 700 K and <7% zinc oxides might be reduced to their metal phase above 1000 K. As known, Zn 2+ cannot be reduced by H 2 due to the positive free Gibbs energy [29] . However, the reduction may proceed if H 2 is split into hydrogen atoms or alloy phase with other metals like Cu is formed [30] . Furthermore, the spinel structure of ZnAlO x has been proved to be more durable under H 2 reduction [31] . As a result, we consider that it is not zinc metal but Zn 2+ in ZnAlO x activates CO 2 hydrogenation reactions in this study. For a long time, the debate about the role of zinc species in industrial Cu/ZnO/Al 2 O 3 catalysts for methanol synthesis has always existed. ZnO in Cu/ZnO/Al 2 O 3 was not reckoned as catalytic centers but structural promoter or others [32] , [33] . However, our results prove that in the absence of Cu species, ZnAlO x can also convert CO 2 into MeOH and derived DME. The FT-IR spectra of catalysts after 2,6-di-tert-butyl-pyridine absorption (DTBPy-FTIR) are exhibited in Fig. 4d . DTBPy-FTIR was usually utilized to investigate the external surface Brønsted acid sites because the kinetic diameter (10.5 Angstrom) of DTBPy is larger than the pore opening (5.5 Angstrom) of H-ZSM-5. The characteristic bands at 3365, 1614 and 1531 cm −1 are attributed to the DTBPy adsorbed on the external surface Brønsted acid sites of H-ZSM-5 zeolite. The negative band at 3616 cm −1 is assigned to the decrease of bridging hydroxyls on the external surface [34] . Surprisingly, these typical bands almost disappeared for the composite catalyst ZnAlO x &H-ZSM-5. It indicates that external Brønsted acid of H-ZSM-5 can be shielded by ZnAlO x after mixing, grinding and pressing under high pressure. The external Brønsted acid has no ability to aromatization but can promote the hydrogenation of unsaturated hydrocarbons to paraffins [15] , [26] , [27] , which is detrimental to the aromatics selectivity. The aromatics or C 2-4 olefins selectivity follows the order ZnAlO x &H-ZSM-5˃   ZnAlO x + H-ZSM-5>ZnAlO x /H-ZSM-5 (Fig. 1b ), whereas the order of C 2-4 paraffins selectivity completely reverses, which verifies this point of view. Fig. 4 Structural characterization of various catalysts. a X-ray diffraction patterns (XRD) of ZnAlO x . b High-resolution transmission electron microscopy (TEM) image of ZnAlO x . Scale bar: 10 nm. c H 2 -TPR profiles. The relative intensity was normalized by weight. The relative intensity of the standard sample Ag 2 O was divided by 50. d FTIR subtraction spectra relative to adsorption of DTBPy Full size image Operando DRIFT study The operando diffuse reflectance infrared Fourier transform spectroscopy (DRIFTS) of CO 2 hydrogenation over ZnAlO x at 593 K and 0.1 MPa are explored. It is obvious from Supplementary Fig. 12 that absorbed surface formate species were first formed, then, absorbed surface methoxy species were generated by hydrogenation of formate species. As presented in Fig. 5 , compared to DRIFTS of CO 2 hydrogenation over ZnAlO x , the bands for surface formate (1620, 1375 and 2910 cm −1 ) and methoxy (2940 and 2840 cm −1 ) species [35] , [36] over ZnAlO x &H-ZSM-5 are sharply weakened, which suggests that these active surface species over ZnAlO x were converted by H-ZSM-5. Combined the catalytic results in Fig. 1a with DRIFTS results discussed above, we propose a mechanism for CO 2 hydrogenation to aromatics over ZnAlO x &H-ZSM-5. First, surface formate species on ZnAlO x was hydrogenated to form surface methoxy species; then, intermediates including MeOH and DME produced from the dissociation of methoxy species were spread to H-ZSM-5 to synthesize olefins intermediates; finally, transformation of olefins to aromatics consecutively take place in the micropores of H-ZSM-5. Furthermore, compared to CO 2 hydrogenation over ZnAlO x , CO hydrogenation generates much less surface formate species. 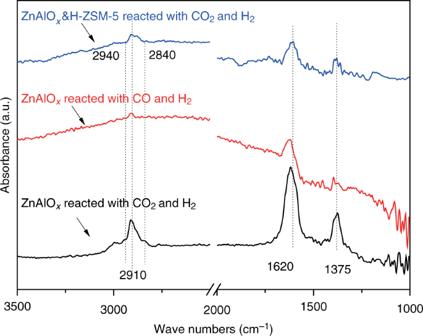Fig. 5 OperandoDRIFT spectra over various catalysts. Conditions: 593 K, 0.1 MPa. CO2&H2refers to the mixed gas of H2/CO2/Ar = 3/1/0.2; CO&H2refers to the mixed gas of H2/CO/Ar = 3/1/0.2 That is to say, more active metal species sites of ZnAlO x are utilized to activate H 2 during CO hydrogenation, so that higher C 2-4 paraffins but lower aromatics are obtained in Supplementary Figure 5 because hydrogenation reactions of intermediates like olefins are enhanced. From Supplementary Fig. 13 , we believe that CO 2 hydrogenation cannot proceed over H-ZSM-5. Some evidences were put forward by Jiao et al. [14] , [17] , [20] to support the ketene intermediate mechanism for STO or STA reactions over oxides/zeolites composite catalysts, however, we consider that this mechanism does not work in CO 2 hydrogenation over ZnAlO x &H-ZSM-5 due to very low concentration of CO in the reaction process. Fig. 5 Operando DRIFT spectra over various catalysts. Conditions: 593 K, 0.1 MPa. CO 2 &H 2 refers to the mixed gas of H 2 /CO 2 /Ar = 3/1/0.2; CO&H 2 refers to the mixed gas of H 2 /CO/Ar = 3/1/0.2 Full size image In summary, composite catalyst of ZnAlO x with a nano-scaled spinel structure and H-ZSM-5 exhibits an excellent performance for CO 2 hydrogenation to aromatics. The selectivity of aromatics (excluding CO) reaches as high as 73.9% with 9.1% CO 2 conversion and 0.4% CH 4 selectivity. Increasing H 2 /CO 2 ratio or introducing CO can effectively suppress RWGS reaction without obviously weakening aromatization. The composite catalyst containing Si-H-ZSM-5 presents higher p -xylene, ethylene and propylene selectivity. It is not zinc metal but Zn 2+ in ZnAlO x activates CO 2 hydrogenation. The shield of the external Brønsted acid of H-ZSM-5 by ZnAlO x is beneficial to aromatization. MeOH, DME and olefins are acted as reaction intermediates. CO 2 hydrogenation over ZnAlO x &H-ZSM-5 shows much higher aromatics selectivity than CO hydrogenation because the former reaction generates more formate species on ZnAlO x surface so that less metal species sites are left for hydrogenation of unsaturated intermediates like olefins. ZnAlO x &H-ZSM-5 suggests a promising application in manufacturing aromatics from CO 2 and H 2 . Catalyst preparation ZnAlO x oxide was prepared by a conventional co-precipitation method. Typically, solution A was made by 59.5 g Zn(NO 3 ) 2 6H 2 O and 75.0 g Al(NO 3 ) 3 9H 2 O dissolved in 150 ml deionized water and solution B was prepared by 23.5 g (NH 4 ) 2 CO 3 dissolved in 150 ml deionized water. Solutions A and B were dividedly added into one beaker by two peristaltic pumps with constant pH of 7.1–7.3 at 343 K under continuous stirring for 0.5 h, then followed by aging for 3 h at the same temperature. After filtered and washed by 200 ml deionized water for three times, the obtained mixture was dried at 373 K overnight and then calcined at 773 K for 4 h. Commercial Na-ZSM-5 zeolite was supplied from Zhongke New Catalytic Technology Company, China. Na-ZSM-5 zeolites were transformed into NH 4 -ZSM-5 by exchanging 50 g Na-ZSM-5 with 0.5 l NH 4 NO 3 (1 mol l −1 ) aqueous solution at 353 K for 2 h, followed by filtration and washing with deionized water. After repeating the exchanging process for three times, the resultant samples were dried overnight at 373 K, followed by calcination at 823 K for another 4 h in air to obtain the H-ZSM-5 zeolite. Si-H-ZSM-5 zeolite was prepared by tetraethoxysilane (TEOS) modification. In brief, an organic solution was firstly made by 11.5 g TEOS mixed with 5 ml cyclohexane; then 10.0 g H-ZSM-5 was added into this solution, impregnated for 24 h at room temperature; after that, organic solvent was removed by evaporation at 353 K and the resultant powder was dried overnight at 373 K, followed by calcination at 823 K for another 4 h in air. After repeating the procedure above for twice, the Si-H-ZSM-5 was obtained. The composite catalysts were typically prepared by physical mixing. Unless specially stated, the weight ratio of oxides and zeolites was 1:1. For preparation of the composite catalyst ZnAlO x &H-ZSM-5, ZnAlO x oxide and H-ZSM-5 zeolite were grinded in an agate mortar for 4 min, pressed under 40 MPa and granulated into the required size in the range of 0.4–0.8 mm. Catalytic tests Catalytic reaction experiments in Fig. 1 and Supplementary Figure 2 and 3 were performed in a 16-channel continuous flow fixed-bed stainless steel reactor (from Yashentech Corporation, Shanghai, China) with an 8.3 mm inner diameter for each channel. The inlet gas flow and composition along with the reaction temperature and pressure for each channel were identical. All the reaction products were kept in the gas phase and analyzed online by two gas chromatographs (Aglient 7890A) equipped with a HP-PLOT/Q capillary column connected to a flame ionization detector (FID) and a TDX-1 column (produced from DICP) connected to a thermal conductivity detector (TCD). CH 4 was taken as a reference bridge between FID and TCD. Ar was used as an inner standard. The CO 2 conversion and the CO selectivity, hydrocarbons (C n H m ), MeOH and DME selectivity among the carbon products without CO (including C n H m , MeOH and DME) were calculated with the followed equations. CO_2 conversion = ( CO_2in - CO_2out)/( CO_2in) × 100%
 (1) CO 2in : moles of CO 2 at the inlet; CO 2out : moles of CO 2 at the outlet; 
    CO selectivity = CO_out/( CO_2in - CO_2out) × 100%
 (2) CO out : moles of CO at the outlet; 
    [ ;                                                      C_nH_m selectivity = N_CnHm/( total carbon atoms of. ;                                                     ;                                                                        . products detected by FID) × 100%;                                                     ;                                                        MeOH selectivity = N_MeOH/( total carbon atoms of. ;                                                     ;                                                                        . products detected by FID) × 100%;                                                     ;                                                         DME selectivity = N_DME/( total carbon atoms of . ;                                                     ;                                                                        . products detected by FID) × 100% ]
 N C n H m : carbon atoms number of C n H m ; N Me6OH : carbon atoms number of MeOH; N DME : carbon atoms number of DME. Other catalytic reaction experiments were performed in a typical fixed-bed stainless steel reactor with 8 mm inner diameter. All products were analyzed online by two tandem gas chromatographs. One is Agilent 7890A equipped with a HP-PLOT/Q capillary column connected to FID and a TDX-1 column connected to TCD. The other one is Agilent 6890N equipped with a HP-FFAP capillary column connected to FID and a Porapak Q column connected to TCD. The detailed analysis for aromatics such as ethylbenzene, p -xylene, m -xylene and o -xylene is dependent on HP-FFAP capillary column.